Did diamond-bearing orangeites originate from MARID-veined peridotites in the lithospheric mantle? Kimberlites and orangeites (previously named Group-II kimberlites) are small-volume igneous rocks occurring in diatremes, sills and dykes. They are the main hosts for diamonds and are of scientific importance because they contain fragments of entrained mantle and crustal rocks, thus providing key information about the subcontinental lithosphere. Orangeites are ultrapotassic, H 2 O and CO 2 -rich rocks hosting minerals such as phlogopite, olivine, calcite and apatite. The major, trace element and isotopic compositions of orangeites resemble those of intensely metasomatized mantle of the type represented by MARID (mica-amphibole-rutile-ilmenite-diopside) xenoliths. Here we report new data for two MARID xenoliths from the Bultfontein kimberlite (Kimberley, South Africa) and we show that MARID-veined mantle has mineralogical (carbonate-apatite) and geochemical (Sr-Nd-Hf-O isotopes) characteristics compatible with orangeite melt generation from a MARID-rich source. This interpretation is supported by U-Pb zircon ages in MARID xenoliths from the Kimberley kimberlites, which confirm MARID rock formation before orangeite magmatism in the area. Orangeites (previously known as Group-II kimberlites) are H 2 O- and CO 2 -rich peralkaline ultrapotassic igneous rocks [1] . Initially considered to be a variety of archetypal (or Group-I) kimberlite, orangeites are now recognized as a distinct magma type, based on their unique mineralogy, mineral chemistry, bulk-rock major and trace element concentrations and isotopic composition [1] , [2] , [3] . Orangeites are widespread in southern Africa with more than 200 known occurrences recognized [1] , [2] , but similar rocks have also been identified in Australia [4] , India [5] , [6] , Russia and Finland [7] . In this regard, Mitchell [8] proposed that orangeites from the Kaapvaal craton (southern Africa) may be local variants of global lamproite-like ultrapotassic magmatism, with all these melts derived from metasomatized lithospheric mantle. Like kimberlites, orangeites occur as small pipes (<2 km in diameter), sills and dykes and are hybrid rocks consisting of mantle-derived xenoliths (that is, rocks fragments) and xenocrysts (including diamonds) set in a matrix of magmatic origin [1] . The magmatic mineralogy is dominated by phlogopite with subordinate olivine (partly xenocrystic), carbonates, apatite and clinopyroxene (not always present), and lesser spinel, perovskite and exotic phases such as REE-phosphates, K-Ba titanates and K-richterite in more evolved varieties [1] . Orangeites are extremely enriched in mantle incompatible elements, particularly LILE (K, Rb, Ba, Sr), Th, U, Pb and LREE [9] , which indicates derivation from partial melting of a metasomatized mantle source. However, their high Mg# (=Mg/(Mg+Fe 2+ )) and compatible element content (for example, Ni, Cr) suggests equilibration with refractory peridotitic mantle that experienced extensive partial melting early in its history [10] . Therefore, orangeite melts appear to have originated from a refractory mantle that experienced subsequent metasomatism by H 2 O/CO 2 -rich fluids/melts enriched in incompatible elements. A number of upper mantle xenolith types entrained by kimberlite and orangeite magmas exhibit these characteristics (see, for example, refs 11 , 12 , 13 ), which supports the widely held hypothesis that orangeite melts are sourced from the metasomatized mantle lithosphere [1] , [9] , [10] , [14] , [15] . This interpretation is also consistent with Sr-Nd isotope data, which indicate a long history of lithospheric mantle enrichment for the orangeite source (that is, radiogenic Sr and unradiogenic Nd isotopes) [3] , [16] . Note that this hypothesis contrasts with an asthenospheric (that is, sub-lithospheric) origin for kimberlites favoured by many authors (see, for example, refs 3 , 16 ). Despite a general consensus on the location of the orangeite source in the lithospheric mantle, considerable uncertainty remains regarding the exact composition of this source. Compositions proposed include phlogopite-carbonate harzburgite [14] , [17] , phlogopite-diopside garnet-bearing peridotite [9] , [15] and peridotite with veins of phlogopite, K-richterite, apatite, carbonates and diopside [1] . It is noteworthy that the veined peridotite composition proposed by Mitchell [1] is very similar to that of the MARID (mica-amphibole-rutile-ilmenite-diopside) suite of mantle xenoliths [18] ; the only notable differences are the presence of Ti-phases and apparent absence of carbonates in MARID rocks. MARID rocks have been transported from the lithospheric mantle to the Earth’s surface by kimberlite, orangeite and lamprophyre magmas from various localities worldwide [18] , [19] , [20] , [21] , [22] . MARID rocks represent an extreme example of mantle metasomatism because of their exceptional enrichment in alkalis, LREE, HFSE (for example, Ti, Zr, Nb) and volatile species, primarily H 2 O (ref. 19 ). For this reason, MARID rocks have been frequently invoked to account for the origin of alkali-rich mafic-ultramafic magmas [23] , [24] , [25] , [26] , with the notable exception of orangeites. Sweeney et al. [27] noted that the bulk major element composition of MARID rocks could be obtained by subtracting the composition of olivine and carbonates from a bulk orangeite composition. In addition, the Sr and Nd isotopic composition of several MARID rocks overlap with the field defined by orangeites [19] . It is therefore possible that a MARID-veined peridotitic mantle could represent the source of orangeite melts. To test this hypothesis, we have examined the composition of primary mineral inclusions in MARID phases and determined the mineral major and trace element concentrations, clinopyroxene Sr-Nd-Hf isotope ratios and zircon U-Pb-Hf-O isotopic compositions for two MARID samples from the Bultfontein kimberlite (Kimberley, South Africa; Fig. 1 ). The Kimberley area is unique because it hosts kimberlites ( ∼ 81–95 Myr ago [16] , [28] , [29] , [30] ) that were emplaced after the orangeites of the Barkly West-Boshof district (115–128 Myr ago [29] , [31] ; Fig. 2 ), and the Kimberley kimberlites host a variety of metasomatized mantle xenoliths, which have been extensively studied [11] , [12] , [18] , [19] , [32] , [33] , [34] , [35] , [36] , [37] . Thus, mantle xenoliths entrained by the Bultfontein kimberlite can be considered representative of the same mantle lithosphere that produced the Barkly West-Boshof orangeites. Our study reveals that MARID minerals contain carbonate-rich primary inclusions and have Hf isotopic compositions similar to southern African orangeites. Some MARID zircons show U-Pb ages that predate the emplacement of orangeites and δ 18 O values above the mantle range. Our results, combined with existing data, confirm that a MARID-veined peridotitic mantle represents a suitable source for orangeite melts. 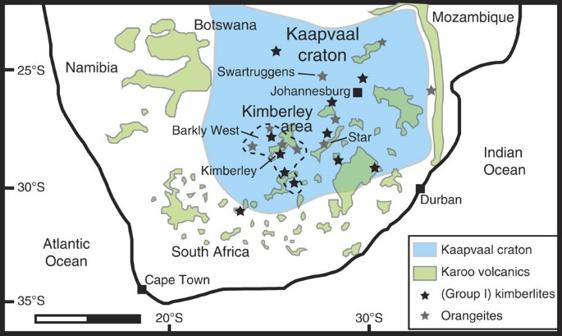Figure 1: Schematic map of southern Africa showing the location of the Kimberley area (modified from Giulianiet al.37). The estimated boundaries of the Kaapvaal craton, the position of major kimberlite and orangeite intrusions around Kimberley and of major outcrops of Karoo igneous rocks are also shown. Scale bar, 500 km. Figure 1: Schematic map of southern Africa showing the location of the Kimberley area (modified from Giuliani et al. [37] ). The estimated boundaries of the Kaapvaal craton, the position of major kimberlite and orangeite intrusions around Kimberley and of major outcrops of Karoo igneous rocks are also shown. Scale bar, 500 km. 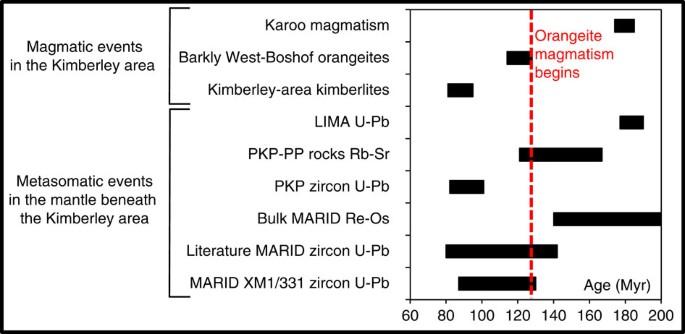Figure 2: Ages of recent magmatic and mantle metasomatic events in the Kimberley area. The emplacement ages of Karoo magmatic rocks (lavas, dykes and sills) are from Jourdanet al.54The Barkly West-Boshof orangeites were emplaced in the Kimberley area at between 114 and 128 Myr ago29,31. The Kimberley-area kimberlites, which include the Kimberley kimberlites and nearby pipes such as Jagersfontein and Kamfersdam, were emplaced between 81 and 95 Myr ago16,28,29,30. U-Pb dating of LIMA (LIndsleyite-MAthiasite) titanates in phlogopite-rich mantle xenoliths from the Bultfontein kimberlite (Kimberley) yielded ages between 177 and 190 Myr ago37. Bulk-rock Rb-Sr analyses of strongly metasomatized, phlogopite±K-richterite-rich peridotite (PP and PKP) xenoliths from the Kimberley kimberlites produced a crude isochron with an age of 144±23 Myr ago70. SHRIMP U-Pb studies of zircon in metasomatized mantle xenoliths from the Kimberley and adjacent Kamfersdam kimberlites produced ages between 81 and 101 for PKP xenoliths32,33,45and 80 and 142 Myr ago for MARID xenoliths32,39,42. The Re-Os model age of a bulk MARID xenolith from the Bultfontein Dumps is 170±30 Myr ago53. U-Pb data for zircons in MARID sample XM1/331 are reported inSupplementary Table 6. Full size image Figure 2: Ages of recent magmatic and mantle metasomatic events in the Kimberley area. The emplacement ages of Karoo magmatic rocks (lavas, dykes and sills) are from Jourdan et al. [54] The Barkly West-Boshof orangeites were emplaced in the Kimberley area at between 114 and 128 Myr ago [29] , [31] . The Kimberley-area kimberlites, which include the Kimberley kimberlites and nearby pipes such as Jagersfontein and Kamfersdam, were emplaced between 81 and 95 Myr ago [16] , [28] , [29] , [30] . U-Pb dating of LIMA (LIndsleyite-MAthiasite) titanates in phlogopite-rich mantle xenoliths from the Bultfontein kimberlite (Kimberley) yielded ages between 177 and 190 Myr ago [37] . Bulk-rock Rb-Sr analyses of strongly metasomatized, phlogopite±K-richterite-rich peridotite (PP and PKP) xenoliths from the Kimberley kimberlites produced a crude isochron with an age of 144±23 Myr ago [70] . SHRIMP U-Pb studies of zircon in metasomatized mantle xenoliths from the Kimberley and adjacent Kamfersdam kimberlites produced ages between 81 and 101 for PKP xenoliths [32] , [33] , [45] and 80 and 142 Myr ago for MARID xenoliths [32] , [39] , [42] . The Re-Os model age of a bulk MARID xenolith from the Bultfontein Dumps is 170±30 Myr ago [53] . U-Pb data for zircons in MARID sample XM1/331 are reported in Supplementary Table 6 . Full size image Sample descriptions MARID xenolith samples XM1/331 and BLFX-3 were collected from the Bultfontein Dumps, which contain waste material predominantly from mining of the Bultfontein kimberlite. 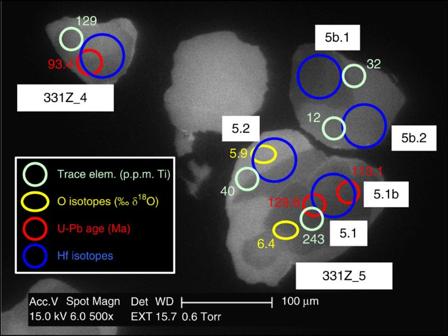Figure 6: CL SEM image of zircon grain in MARID sample XM1/331. Also shown are the areas analysed for trace elements, O, U-Pb and Hf isotopes together with Ti concentrations (p.p.m.), δ18O (‰) values and U-Pb ages (Myr ago). The Bultfontein kimberlite is part of the Kimberley cluster of kimberlites ( Fig. 1 ), which have been classified as archetypal kimberlites based on their mineralogy and Sr-Nd isotopic signature [3] . The Kimberley kimberlites were emplaced between ∼ 81 and 90 Myr ago, based on Rb-Sr phlogopite [28] , [38] and U-Pb perovskite geochronology [30] ( Fig. 2 ). MARID xenoliths are relatively common in the Kimberley kimberlites [12] , [18] , [19] , [35] , [39] , [40] . The two samples studied here exhibit coarse-grained foliated textures, with compositional banding related to the preferential concentrations of K-richterite and phlogopite in discrete layers ( Fig. 3 ), a common feature of MARID rocks [18] , [19] . Clinopyroxene in textural equilibrium with phlogopite and K-richterite occurs in sample XM1/331, but is absent in sample BLFX-3—again this is not unusual for MARID samples [18] . Oxide minerals, including rutile in sample XM1/331 and ilmenite in sample BLFX-3, are widespread and account for up to ∼ 5 vol% of the xenoliths. Zircon grains are locally abundant in sample XM1/331, where they occur as isolated grains or clusters of grains included in, or interstitial to, K-richterite and rutile ( Fig. 4 ). K-richterite inclusions are frequently observed in zircons ( Fig. 4d ). 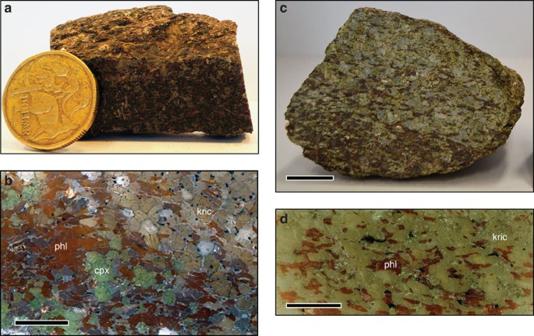No zircons were observed in sample BLFX-3. Figure 3: Photographs of off-cuts and thin-section scans of MARID samples. Samples XM1/331 (a,b) and BLFX-2 (c,d) show foliated texture due to preferential concentration of K-richterite (kric) and phlogopite (phl) in discrete layers. Note that clinopyroxene (cpx) only occurs in sample XM1/331. Coin diameter, 2.4 cm. Scale bars inb,c,dare 0.5, 2 and 1 cm, respectively. Figure 3: Photographs of off-cuts and thin-section scans of MARID samples. Samples XM1/331 ( a , b ) and BLFX-2 ( c , d ) show foliated texture due to preferential concentration of K-richterite (kric) and phlogopite (phl) in discrete layers. Note that clinopyroxene (cpx) only occurs in sample XM1/331. Coin diameter, 2.4 cm. 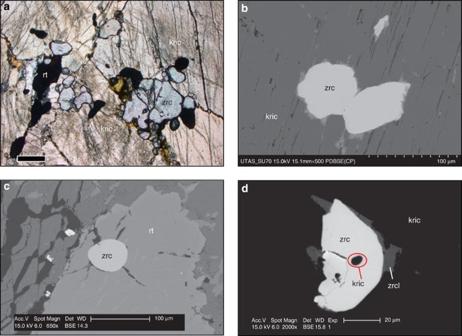Scale bars in b , c , d are 0.5, 2 and 1 cm, respectively. Figure 4: Images of zircon grains in MARID sample XM1/331. Optical photomicrograph of cluster of zircon (zrc) grains interstitial to K-richterite (kric) (a; scale bar, 0.5 mm) and back-scattered electron (BSE) SEM images of zircon grains included in K-richterite (b,d) and rutile (rt) (c). Ind, note the K-richterite inclusion in zircon, which is rimmed by zirconolite (zrcl). Full size image Figure 4: Images of zircon grains in MARID sample XM1/331. Optical photomicrograph of cluster of zircon (zrc) grains interstitial to K-richterite (kric) ( a ; scale bar, 0.5 mm) and back-scattered electron (BSE) SEM images of zircon grains included in K-richterite ( b , d ) and rutile (rt) ( c ). In d , note the K-richterite inclusion in zircon, which is rimmed by zirconolite (zrcl). Full size image Pervasive carbonate-rich veins traverse both samples, a feature that is common to many other documented MARID xenoliths [18] , [19] . MARID minerals in contact with these veins occasionally display thin (<10 μm) overgrowths and reaction rims, including clinopyroxene on K-richterite and baddeleyte plus zirconolite rimming zircon ( Fig. 4d ). The formation of these veins is attributed to reaction with late-stage fluids from the entraining kimberlite magma [18] , [19] . Primary inclusions in MARID minerals In both xenoliths, K-richterite hosts inclusions of the other major mineral constituents (for example, phlogopite, clinopyroxene, rutile and zircon in K-richterite from sample XM1/331), whereas phlogopite contains occasional inclusions of K-richterite and the dominant oxide phase (that is, rutile or ilmenite). However, neither K-richterite nor phlogopite is ideal for studying their primary inclusion mineralogy, particularly with respect to minerals (for example, carbonates) readily modified by late-stage fluids, because of their strong cleavage. Conversely, clinopyroxene and ilmenite appear to be more resistant to reaction with late-stage mantle and/or crustal fluids and preserve their original primary inclusion assemblages. Clinopyroxene from sample XM1/331 hosts abundant small (<10 μm), primary carbonate-rich inclusions with irregular to amoeboid shapes ( Fig. 5a and Supplementary Figs 1 and 2 ). The inclusions are distributed heterogeneously and are enriched in alkali carbonates (that is, shortite Na 2 Ca 2 (CO 3 ) 3 , zemkorite (Na,K) 2 Ca(CO 3 ) 2 and Na-K-rich calcite), Na-rich fluoroapatite, abundant phlogopite (and tetraferriphlogopite), K-richterite and Fe-Ti oxides, but also host minor strontian barite. Similar inclusions occur in mantle polymict breccia xenoliths [34] , [36] , although the latter are more enriched in carbonates over silicate phases. Rare primary carbonate-rich inclusions were also documented in the cores of ilmenite grains from sample BLFX-3. These inclusions are elongated and are up to 15 μm in size. They are composed of dolomite with variable Na 2 O and K 2 O concentrations and, in one instance, zemkorite ( Fig. 5b and Supplementary Figs 1 and 2 ). 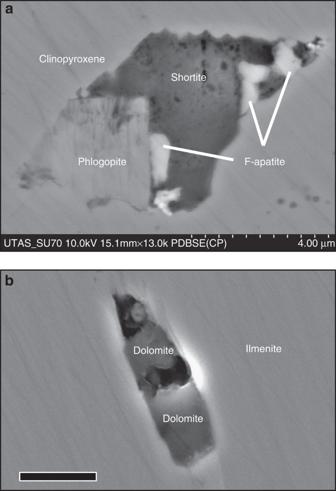Inclusions of Ni-Fe sulphides also occur in ilmenite from sample BLFX-3. Figure 5: Back-scattered electron SEM images of primary carbonate-rich inclusions in MARID minerals. (a) Inclusion of shortite (Na2Ca2(CO3)3), tetraferriphlogopite and Na-rich fluoroapatite in clinopyroxene grain of sample XM1/331; (b) inclusion of alkali-bearing dolomite in ilmenite grain of sample BLFX-3 (scale bar, 5 μm). Additional SEM images are inSupplementary Figs 1 and 2. Figure 5: Back-scattered electron SEM images of primary carbonate-rich inclusions in MARID minerals. ( a ) Inclusion of shortite (Na 2 Ca 2 (CO 3 ) 3 ), tetraferriphlogopite and Na-rich fluoroapatite in clinopyroxene grain of sample XM1/331; ( b ) inclusion of alkali-bearing dolomite in ilmenite grain of sample BLFX-3 (scale bar, 5 μm). Additional SEM images are in Supplementary Figs 1 and 2 . Full size image Major and trace element composition of MARID minerals The major oxide compositions of K-richterite, clinopyroxene, phlogopite, ilmenite and rutile in the two MARID xenoliths are reported in Supplementary Table 1 , with trace element compositions listed in Supplementary Tables 2 and 3 . Supplementary Figs 3 and 4 show that these compositions are broadly in the range of minerals from previously studied MARID rocks [12] , [18] , [19] , [41] . Zircon trace elements and U-Pb-Hf-O isotopic compositions Zircons from sample XM1/331 are variable in size (up to ∼ 0.5 mm), with rounded to irregular shapes ( Figs 4 and 6 ), which are typical of zircons formed in mantle rocks. Scanning electron microscope (SEM) cathodoluminescence (CL) imaging reveals that these zircons have complex textures, with darker CL areas partially enclosed and traversed by domains with brighter CL response ( Fig. 6 and Supplementary Fig. 5 ; see also refs 39 , 40 , 42 ). Bright CL domains have low trace element contents (ΣREE≤43 p.p.m. ; Y≤52 p.p.m. ; U≤36 p.p.m.) and the highest Yb/Sm ratios ( Supplementary Fig. 6 ). Such compositions are typical of zircon megacrysts in kimberlites [43] . Dark CL domains have higher trace element contents (ΣREE=68–414 p.p.m. ; Y=78–501 p.p.m. ; U=44–155 p.p.m. ; Supplementary Table 4 ), similar to compositions of zircons in lamproites and carbonatites [43] ( Supplementary Fig. 7 ). Figure 6: CL SEM image of zircon grain in MARID sample XM1/331. Also shown are the areas analysed for trace elements, O, U-Pb and Hf isotopes together with Ti concentrations (p.p.m. ), δ 18 O (‰) values and U-Pb ages (Myr ago). Full size image In situ SHRIMP U-Pb dating of zircons from xenolith XM1/331 produced variable 206 Pb/ 238 U ages ranging from 86.6±1.4 to 129.8±2.0 (2 s.d.) Myr ago ( Fig. 2 and Supplementary Table 6 ; see Methods for analytical details). There is no correlation between grain size and U-Pb age indicating that the age variation is not due to diffusive loss of radiogenic Pb. The 207 Pb/ 206 Pb versus 238 U/ 206 Pb Concordia diagram shows that the majority of analyses (18/23) plot along a regression line corresponding to a lower intercept age of 89.6±1.2 Myr ago (2 s.d. ; mean square weighted deviation (MSWD)=1.09— Supplementary Fig. 8 ). The weighted 206 Pb/ 238 U age for these analyses is 90.1±0.6 Myr ago ( n =16/18; MSWD=2.0). The remaining five analyses correspond to some of the dark CL areas (see, for example, Fig. 6 ) and yielded ages between 98.1±2.1 and 129.8±2.0 Myr ago ( Supplementary Figs 5 and 6 ). This age range is comparable to the previous U-Pb ages for zircons from MARID xenoliths (80–142 Myr ago [32] , [39] , [42] , [44] ) and PKP (phlogopite+K-richterite peridotite) rocks (82–101 Myr ago [32] , [33] , [45] ) from the Kimberley area ( Fig. 2 ). Oxygen isotope ratios in zircons from xenolith XM1/331 (δ 18 O=5.3–6.6‰; Fig. 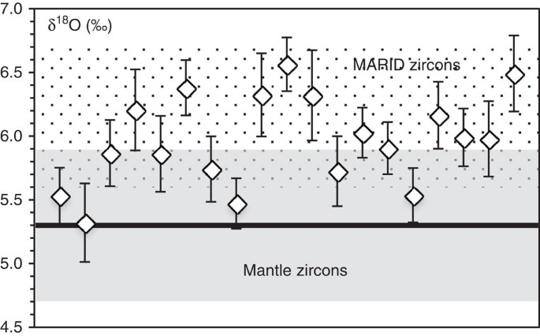Figure 7: Oxygen isotopic composition of zircon grains in MARID sample XM1/331. The compositions are reported as ‰ δ18O relative to SMOW. Error bars are 2 s.d. MARID zircons refer to the grains recently analysed by Konzettet al.40in another xenolith from the Bultfontein kimberlite. Mantle zircons δ18O=5.3±0.6‰ (ref.46) (2 s.d.). 7 and Supplementary Table 7 ), which was measured by ion microprobe (see Methods), show greater variation than is accountable from analytical uncertainty alone (±0.3‰, 2 s.d.). This is supported by the high MSWD (8.9) of the weighted average of these results (5.94±0.17‰; n =18; 2 s.e.). Figure 7 shows that at least seven analyses plot above the field of mantle zircons (δ 18 O=5.3±0.6‰ (ref. 46 ). It is notable that the δ 18 O values of the XM1/331 zircons are not correlated with the CL response, U-Pb age or trace element concentration of analysed areas ( Supplementary Figs 5, 6 and 9 ). Konzett et al. [40] recently reported a very similar range of δ 18 O values (5.6–6.7‰; Fig. 7 ) for zircon grains in another MARID xenolith from Bultfontein. Figure 7: Oxygen isotopic composition of zircon grains in MARID sample XM1/331. The compositions are reported as ‰ δ 18 O relative to SMOW. Error bars are 2 s.d. MARID zircons refer to the grains recently analysed by Konzett et al. [40] in another xenolith from the Bultfontein kimberlite. Mantle zircons δ 18 O=5.3±0.6‰ (ref. 46 ) (2 s.d.). 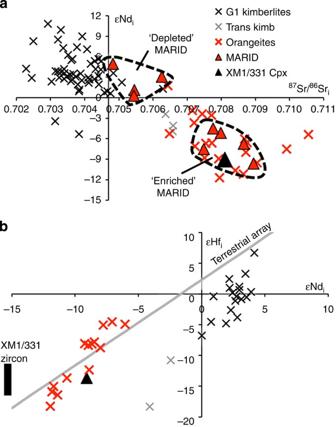Figure 8: Sr-Nd-Hf isotopic composition of MARID minerals and southern African orangeites and kimberlites. (a)87Sr/86SrivsɛNdi(corrected fort=90 Myr ago, that is, approximate age of the entraining Kimberley kimberlites) of XM1/331 clinopyroxene and minerals (apatite, clinopyroxene, K-richterite) in previously analysed MARID xenoliths from the Kimberley area19,38; and initial87Sr/86Sr and ɛNd values of <250 Myr ago archetypal kimberlites, transitional kimberlites and orangeites from southern Africa16. (b) ɛNdivs ɛHfiof XM1/331 clinopyroxene and southern African archetypal kimberlites, transitional kimberlites and orangeites15,49. ɛHf(90Ma)range of XM1/331 zircon is also shown. Terrestrial array from Vervoortet al.48 Full size image 176 Hf/ 177 Hf ratios of the XM1/331 zircons, as measured in situ by LA–MC–ICP–MS (see Methods), vary between 0.28218 and 0.28241 (36 analyses on 18 grains; Supplementary Table 8 ). Correction to 90 Myr ago yields ɛHf (90Ma) values in the range −19.4 to −11.6. Removal of one obvious outlier (spot 331A_2.2) reduces this range to −16.6 to −11.6, with an average of −13.8±2.6 (2 s.d.). This range only marginally exceeds the analytical reproducibility, estimated at ∼ ±2 ɛHf units, which contrasts with the large variability in trace element concentrations, U-Pb and O isotopic systematics. The homogeneity is attributed to slower Hf diffusion in zircon compared to O, Pb and REEs [47] . Clinopyroxene Sr-Nd-Hf isotopes Solution ICP–MS isotopic analyses of clinopyroxene grains from xenolith XM1/331 yielded the following present-day 87 Sr/ 86 Sr, 143 Nd/ 144 Nd and 176 Hf/ 177 Hf (±2 s.e.) ratios: 0.708135±0.000018, 0.512117±0.000008, 0.282359±0.000009 ( Table 1 ; see Methods for analytical details). Correction for radiogenic ingrowth since emplacement of the Bultfontein kimberlite at ∼ 84 Myr ago [38] yields 87 Sr/ 86 Sr i =0.708105±0.000018, ɛNd i =−9.1±0.3 and ɛHf i =−13.7±0.5. The ɛHf i value is identical to that of zircon from the same sample, and is equivalent to an offset from the global Hf-Nd isotope array [48] of ΔɛHf=−3.3 ( Fig. 8 ). These values are also similar to ɛHf (84Ma) values (−16.7 to −17.8) reported for zircon grains in another MARID xenolith from the Bultfontein kimberlite by Choukroun et al. [44] The clinopyroxene Sr-Nd isotopic composition is within the ‘enriched’ field of MARID minerals ( Fig. 8a ). Table 1 Solution-mode Sr-Nd-Hf isotope results for clinopyroxene in MARID sample XM1/331. Full size table Figure 8: Sr-Nd-Hf isotopic composition of MARID minerals and southern African orangeites and kimberlites. ( a ) 87 Sr/ 86 Sr i vs ɛNd i (corrected for t =90 Myr ago, that is, approximate age of the entraining Kimberley kimberlites) of XM1/331 clinopyroxene and minerals (apatite, clinopyroxene, K-richterite) in previously analysed MARID xenoliths from the Kimberley area [19] , [38] ; and initial 87 Sr/ 86 Sr and ɛNd values of <250 Myr ago archetypal kimberlites, transitional kimberlites and orangeites from southern Africa [16] . ( b ) ɛNd i vs ɛHf i of XM1/331 clinopyroxene and southern African archetypal kimberlites, transitional kimberlites and orangeites [15] , [49] . ɛHf (90Ma) range of XM1/331 zircon is also shown. Terrestrial array from Vervoort et al. [48] Full size image Although MARID rocks have never been invoked as the mantle source for orangeite magmas, links between MARID rocks and orangeites have long been recognized and include: MARID xenoliths and related xenocrysts have been recovered from orangeite intrusions, including Star, Swartruggens and those in the Barkly West-Boshof district [15] , [18] , [19] (South Africa; Fig. 1 ); MARID and orangeite rocks have similar bulk major element compositions once olivine and carbonate components have been subtracted from orangeite compositions [27] ; calculated REE patterns of melts in equilibrium with MARID diopside resemble those of orangeite rocks [12] ; zircon U-Pb ages of some MARID xenoliths from the Kimberley area [39] , [42] overlap the timing of nearby Barkley West-Boshof orangeite magmatism ( Fig. 2 ); the Sr-Nd isotopic compositions of orangeites largely overlap the ‘enriched MARID’ field and extend towards (and, a single analysis, into) the field of ‘depleted MARID’ ( Fig. 8a ). It is noteworthy that the analysed MARID samples in the depleted field were entrained by archetypal kimberlite magmas and, to some extent, could be isotopically re-equilibrated with and/or contaminated by the entraining kimberlite. These observations and inferences have been used to argue that MARID rocks were produced by orangeite melts at lithospheric mantle conditions [12] , [27] , [39] . In the following discussion, we provide additional constraints supporting a genetic link between MARID assemblages and orangeite magmas. However, we also demonstrate that MARID metasomatism in the Kimberley area predates the formation of orangeite melts. Therefore, previous models are untenable and we show that it is more likely that MARID metasomatized mantle was the source for orangeite magmatism. Evidence supporting the origin of orangeites from MARID mantle includes: Hafnium isotopes The Hf isotopic compositions of minerals in MARID sample XM1/331 reflect the proposed MARID-orangeite genetic link. The Nd-Hf isotopic composition of XM1/331 clinopyroxene and the Hf isotopic ratios of MARID zircons analysed in this and a previous study [44] overlap the range of South African orangeites ( Fig. 8b ) including those in the Barkly West-Boshof area [15] , [49] . Oxygen isotopes Schulze et al. [50] suggested that the oxygen isotopic composition of garnet megacrysts in orangeites (δ 18 O=5.59±0.18‰, compared with 5.24±0.15‰ for garnet megacrysts in kimberlites) requires a δ 18 O-rich component in the source of orangeites. Thus, it is noteworthy that several oxygen isotope analyses of MARID zircons analysed in this and a previous study [40] plot above the mantle range ( Figs 6 and 7 ). This suggests that heavy oxygen isotopic compositions could be a characteristic feature of MARID rocks. The formation of zircon rims with depleted trace element contents (megacryst like) and the presence of baddeleyite and zirconolite coronae around XM1/331 zircons ( Fig. 4 ), indicates interaction with fluids/melts after zircon formation. The well-constrained U-Pb age of 90.1±0.6 Myr ago produced from all zircon rims and bright CL areas (plus some dark CL areas; Supplementary Fig. 6 ) suggests that this interaction occurred during the kimberlite magmatic event that affected the Kimberley area at ∼ 81–95 Myr ago ( Fig. 2 ; see also ref. 39 ). Previous oxygen isotope studies of mantle xenoliths in the Kimberley area have reported anomalously low δ 18 O values (<5‰) for minerals that crystallized from, or interacted with, kimberlite-related fluids/melts [51] , [52] . Therefore, interaction with kimberlite-related fluids might be expected to lower the originally high δ 18 O values of the XM1/331 zircons, which is consistent with mantle-like values shown by some of the analyses ( Fig. 7 ). Similarly, the trace element compositional variations shown by XM1/331 zircons ( Supplementary Fig. 7 ) could be explained by mixing between existing, trace element-enriched MARID zircons and trace element-poor domains that formed close to the time of kimberlite magmatism. The lack of systematic correlation between O isotope and trace element compositions (and hence CL response) is probably due to the variable diffusion rates of oxygen compared with the trace elements [47] . In summary, higher-than-mantle δ 18 O values of XM1/331 zircons appear to be an original feature of MARID zircons, whereas lower δ 18 O values probably reflect subsequent interaction with fluids/melts related to the kimberlite magmatic event at ∼ 90 Myr ago. Carbonate-apatite inclusions Additional constraints supporting a genetic link between MARID rocks and orangeites derive from the composition of primary inclusions in MARID minerals. Although the volatile component of orangeites is dominated by H 2 O, the high concentrations of CO 2 and P in orangeite magmas (4.2±2.8 and 1.9±0.8 wt%, respectively) [9] require a source hosting carbonates and phosphates [1] , [17] . In particular, the absence of mantle-derived carbonates (that is, unrelated to late-stage kimberlite or crustal fluids) in MARID rocks represents one of the major compositional differences between MARID rocks and orangeites [27] . The current and previous studies of primary inclusions in MARID minerals have shown that, in addition to typical MARID phases (phlogopite, K-richterite, clinopyroxene, rutile, ilmenite, occasional zircon), apatite is a common included mineral [39] , [40] , [42] . Furthermore, our SEM observations demonstrate that alkali-rich carbonates (for example, shortite, Na-K-bearing dolomite; Fig. 5 ) are also important primary inclusions in MARID minerals. Therefore, it seems likely that carbonates and apatite in MARID rocks were interstitial to the major silicate minerals and were subsequently removed or replaced through interaction with the highly reactive host kimberlite magma or related fluids. There is abundant evidence for the crystallization of serpentine, calcite, phlogopite, sulphates and other volatile-rich minerals in veins traversing MARID rocks, from late-stage kimberlite or crustal fluids during or after xenolith entrainment by kimberlite magmas (this study and refs 12 , 18 , 19 , 35 ). Geochronology The available geochronological data for MARID rocks, the host Kimberley kimberlites and the adjacent Barkly West-Boshof orangeites, support the suggestion of a MARID mantle source for orangeite magmas. U-Pb dating of zircons in MARID xenoliths entrained by the Kimberley kimberlites provides ages as old as ∼ 130 (this study) and ∼ 142 Myr ago [39] . In addition, Pearson et al. [53] reported a Re-Os model age of 170±30 Myr ago for a Kimberley MARID xenolith. These ages extend the timing of MARID metasomatism in the Kimberley region before orangeite magmatism (114–128 Myr ago [29] , [31] ; ‘Barkly West-Boshof orangeites’ in Fig. 2 ). The major thermomagmatic event that affected the Kimberley area before the Barkly West-Boshof orangeite magmatism was the emplacement of Karoo dykes and lavas at ∼ 180 Myr ago [54] , [55] . It is therefore likely that MARID assemblages crystallized from melts produced during the Karoo event, coeval with phlogopite-rich metasomatism in the lithospheric mantle beneath the Kimberley region [37] (‘LIMA U-Pb’ in Fig. 2 ). MARID zircon ages were then partially reset by subsequent geological events. Depth constraints Finally, based on the thermobarometry of entrained xenoliths, it is estimated that orangeite magmas originated from minimum depths of 150–200 km, corresponding to the lower part of the lithospheric mantle in the garnet stability field. Experimental petrology has shown that MARID assemblages are stable to the base of the lithospheric mantle in cold cratons [41] such as the Kaapvaal; this is confirmed by the occurrence of K-richterite+phlogopite inclusions in diamonds [56] . Primitive mantle-normalized trace element patterns for orangeite rocks show characteristic relative depletions in Rb, K, Sr, Nb, Ta and Ti compared with elements of similar incompatibility in mantle peridotites [9] . One explanation for these geochemical features is the occurrence of residual phases in the melt source that concentrated these elements (that is, bulk solid/liquid partition coefficient for these elements >1). The occurrence of residual MARID minerals, such as phlogopite (Rb, K), diopside or K-richterite (Sr) and rutile or ilmenite (Ti, Nb, Ta), in the orangeite source could account for the trace element characteristics of orangeites. This is consistent with experimental results for partial melting of a synthetic Fe-free MARID assemblage at mantle conditions, which showed that diopside, rutile and a K-rich phase (phlogopite or K-richterite) are included in the partial melting residue [57] . In contrast to previous arguments [15] , we propose that the main MARID minerals would persist in the source after low-degree partial melting to produce orangeite melts. In summary, MARID rocks and orangeite magmas share many geochemical (major and trace element) and isotopic (Sr-Nd-Hf-O) features. The occurrence of MARID xenoliths and related xenocrysts in South African orangeites [15] , [18] , [19] coupled with U-Pb dating of MARID zircons (this study and ref. 39 ) and Re-Os dating of a MARID xenolith [53] in the Kimberley area, indicate that MARID rocks were already present in the lithospheric mantle before orangeite magmatism. However, melting of MARID rocks alone fails to explain some geochemical features of orangeites, including their high Mg# ( ∼ 85), Cr and Ni concentrations ( ∼ 2,000 and 1,000 p.p.m., respectively) [9] . These characteristics require the presence of refractory peridotites in the orangeite source and/or assimilation of wall-rock material during magma ascent through the lithospheric mantle. Melting experiments on natural MARID rocks have shown that MARID assemblages have lower melting temperature compared with peridotitic rocks [27] . Partial melting of MARID rocks (possibly in veins) and adjacent refractory peridotites would be consistent with the major (for example, Mg#) and trace element characteristics (for example, relative depletion of Rb, K, Sr, Nb, Ta and Ti) of orangeite magmas. In this regard, the highly fractionated REE patterns of orangeites (that is, (La/Yb) N =168) [9] could be due to either the occurrence of garnet in the peridotite source [9] , [17] , which remains in the partial melting residue, or the LREE-rich composition of the MARID veins. Whereas both MARID veins and peridotitic wall rocks would control the major oxide and compatible trace element (for example, Ni, Cr) composition of the orangeite partial melt, the incompatible trace element and Sr-Nd-Hf isotopic compositions would be governed by the MARID source rocks (see ref. 58 ). The occurrence of carbonates in MARID rocks would also satisfy the condition that orangeite melts are sourced from a carbonated mantle [1] , [14] , [17] . It is concluded that a MARID-veined peridotitic mantle represents the best candidate for the source of orangeite magmas. MARID rocks [18] , [19] , [20] , [21] , [22] and rocks produced by metasomatized lithospheric mantle magmas [8] with features similar to orangeites [1] , [4] , [5] , [6] , [7] have been identified in localities worldwide. It is therefore likely that the genetic relationship that we have established between mantle MARID assemblages and orangeite melts in South Africa can be extended to other continents. SEM study of primary inclusions Initial studies of inclusions in MARID minerals were performed on carbon-coated thin sections using a Philips (FEI) XL30 ESEM TMP, equipped with an OXFORD INCA energy-dispersive X-ray spectrometer (EDS) at the University of Melbourne. More detailed examination of the inclusions was undertaken on thin sections and mineral mounts prepared with liquid hydrocarbons (that is, in the absence of water to preserve water-soluble minerals), using a Hitachi SU-70 field-emission SEM equipped with an OXFORD INCA-XMax80 EDS at the Central Science Laboratory, University of Tasmania (see Giuliani et al. [36] for details of analytical conditions). Major and trace element analyses of mineral phases Electron microprobe analyses of MARID minerals were carried out on thin sections and epoxy mounts, using a Cameca SX50 electron microprobe at the University of Melbourne and employing the same conditions described by Giuliani et al. [36] Trace element abundances in MARID minerals were measured in situ , using an Agilent 7700x quadrupole ICP–MS interfaced with an excimer 193-nm ultraviolet laser ablation probe. Laser ablation conditions were as follows: ablation time of 60 s; fluence ∼ <3 J cm −2 , repetition rate of 5 Hz; standard delay for sample washout of 15 s; longer delay for background measurements (50 s) every five analyses; beam size of 30–42 μm. The synthetic glass NIST612 was used as the calibration material for measurements of K-richterite, clinopyroxene and phlogopite, and 40 Ca (K-richterite and clinopyroxene) and 28 Mg (phlogopite) were the internal standards with Ca and Mg concentrations determined from electron microprobe analyses. For analyses of ilmenite and rutile, we employed BHVO2-G as the calibration material and 49 Ti was the internal standard, whereas NIST610 was used as the calibration material for zircon measurements with Hf as the internal standard. Natural and synthetic glasses NIST610, NIST612, BCR-2-G and BHVO2-G were also analysed as unknowns to verify data integrity ( Supplementary Table 5 ); these glasses yielded results consistent with published values (that is, GeoRem preferred values [59] ). U-Pb and oxygen isotope analyses of zircons Thin-section fragments from sample XM1/331, which contained numerous zircon grains, were cut and encased in epoxy resin. The zircons were then imaged with SEM CL at the University of Melbourne to reveal internal structures. U-Pb age determinations were carried out using a SHRIMP II instrument at the Australian National University. A spot size of ∼ 20 μm was employed. The data were reduced in a manner similar to that described by Williams [60] . The U/Pb ratios and U-Th concentrations were calculated relative to the Temora-2 zircon standard [61] . Pb*/U (where Pb* indicates radiogenic Pb) ratios were calculated by assuming 206 Pb/ 238 U- 207 Pb/ 235 U age concordance ( Supplementary Table 6 ). Age calculations and data representation were accomplished using the Isoplot software [62] . Oxygen isotope analyses of zircons were carried out using the same SHRIMP II instrument and with a similar spot size ( ∼ 20–25 μm). Instrument set-up and the data reduction scheme employed are reported in Ickert et al. [63] The Temora-2 zircon standard was measured together with the unknowns and produced a weighted δ 18 O of 8.22±0.11‰ (2 s.e. ; Supplementary Table 7 ), which is undistinguishable from the accepted value of 8.2‰ (ref. 63 ). Hafnium isotope analyses of zircons In situ Lu–Hf isotopic measurements of the zircon grain were undertaken at the University of Melbourne, using an Nu Plasma multicollector ICP–MS interfaced with an excimer 193 nm ultraviolet laser ablation probe. Laser ablation conditions were as follows: ablation time of 60 s; fluence ∼ <3 J cm −2 , repetition rate of 5 Hz; standard delay of 30 s for sample washout and background measurements; beam size of 55 μm. Raw data were reduced using the Iolite software package [64] . Isobaric interferences of 176 Yb and 176 Lu on 176 Hf were assessed and corrected following the procedure described by Woodhead et al. [65] Plesovice zircon standard [66] was analysed to correct for instrumental drift, whereas Temora-2 and 91500 zircon references [67] were measured as unknowns to assess data quality and returned values ( 176 Hf/ 177 Hf=0.282660±0.000070 ( n =5; 2 s.d.) and 0.282313±0.000040 ( n =3; 2 s.d. ), respectively) within error of the solution values provided by Woodhead and Hergt [67] ( Supplementary Table 8 ). On the basis of the results for standards (this session and long term), analytical reproducibility (external precision) for 176 Hf/ 177 Hf is ∼ ±0.000050 (2 s.d. ), equivalent to ∼ ±1.8 ɛHf units. Sr-Nd-Hf isotope analyses Bulk mineral radiogenic isotope data for XM1/331 clinopyroxene were acquired using two splits of the same separate. For Sr isotope analyses, an 18-mg split was cleaned with nitric acid (1 M, 40 °C, 20 min) and dissolved on a hotplate (HF-HNO 3 and HNO 3 , 100 °C, 3 days). Following equilibration with a 85 Rb- 84 Sr spike, Sr was extracted using EICROM Sr-resin; Rb in the Sr-free eluate was further purified on a 4-ml column of AG50-X8 (100–200) cation resin. For bulk mineral Nd-Hf isotope analyses, a separate split of clinopyroxene (11 mg) was subjected to a relatively harsh leaching protocol (6 M HCl, 60 °C, 45 min; 5% HF, 20 °C, 15 min) [68] to remove kimberlitic contamination from grain surfaces and internal cracks. After repeated rinsing and centrifuging, the sample residue was dissolved in HF-HNO 3 and HNO 3 on a hotplate (100 °C). An ∼ 10% split of the dissolved clinopyroxene residue was used for trace element analysis on an Agilent 7700x quadrupole ICP–MS. USGS basalt BCR-2, analysed in the same batch, yielded results consistent with published values (that is, GeoReM preferred values [59] ). Nd and Hf were extracted from the remaining solution using EICHROM RE- and LN-resins. All isotopic analyses were carried out on an Nu Plasma MC–ICP–MS at the University of Melbourne. Sample solutions were introduced via a low-uptake PFA nebulizer and a CETAC Aridus desolvating system, resulting in sensitivities in the range 80–140 V per p.p.m. 87 Sr/ 86 Sr ratios are reported relative to SRM987=0.710230 and have an internal precision of ±0.000020 (2 σ ). On the basis of the long-term reproducibility for rock standards, the external precisions (2 σ ) are estimated to be: 87 Rb/ 86 Sr 0.5%, 147 Sm/ 144 Nd 2%, 176 Lu/ 177 Hf 2%, 87 Sr/ 86 Sr ±0.000040, 143 Nd/ 144 Nd ±0.000020, 176 Hf/ 177 Hf ±0.000015. ɛNd and ɛHf were calculated for a modern chondritic reservoir with the composition recommended in Bouvier et al. [69] The decay constants used for age corrections are: 87 Rb 1.395 × 10 −11 , 147 Sm 6.54 × 10 −12 and 176 Lu 1.865 × 10 −11 a −1 . How to cite this article : Giuliani, A. et al. Did diamond-bearing orangeites originate from MARID-veined peridotites in the lithospheric mantle? Nat. Commun. 6:6837 doi: 10.1038/ncomms7837 (2015).